Solution-state conformation and stoichiometry of yeast Sir3 heterochromatin fibres Heterochromatin is a repressive chromatin compartment essential for maintaining genomic integrity. A hallmark of heterochromatin is the presence of specialized nonhistone proteins that alter chromatin structure to inhibit transcription and recombination. It is generally assumed that heterochromatin is highly condensed. However, surprisingly little is known about the structure of heterochromatin or its dynamics in solution. In budding yeast, formation of heterochromatin at telomeres and the homothallic silent mating type loci require the Sir3 protein. Here, we use a combination of sedimentation velocity, atomic force microscopy and nucleosomal array capture to characterize the stoichiometry and conformation of Sir3 nucleosomal arrays. The results indicate that Sir3 interacts with nucleosomal arrays with a stoichiometry of two Sir3 monomers per nucleosome. We also find that Sir3 fibres are less compact than canonical magnesium-induced 30 nm fibres. We suggest that heterochromatin proteins promote silencing by ‘coating’ nucleosomal arrays, stabilizing interactions between nucleosomal histones and DNA. Eukaryotic genomes are assembled into a complex assembly of proteins and DNA known as chromatin. The basic unit of chromatin is the nucleosome, which consists of 147 base pairs of DNA wrapped approximately twice around an octamer of histones containing two copies each of histones H2A, H2B, H3 and H4 (ref. 1 ). Within the nucleus, long linear arrays of nucleosomes are organized into two functionally distinct compartments, termed euchromatin and heterochromatin. Euchromatic regions are often referred to as ‘active’ chromatin, as they harbour transcriptionally active gene loci, whereas heterochromatin contains ‘inactive’ chromatin domains that are generally repressive for transcription and typically localize to the nuclear periphery [2] . Heterochromatin is required for the organization and function of centromeres [3] , as well as the protection of telomeres [4] . In addition, heterochromatin protects genome integrity by repressing the transposition of abundant transposable elements and by preventing extensive or illicit recombination between dispersed repetitive DNA elements [5] , [6] . Although heterochromatin assembly is known to require interactions between heterochromatin-specific architectural proteins and nucleosomes, the way in which these proteins organize a nucleosomal array into the overall repressive conformation remains poorly understood [7] , [8] , [9] , [10] . In Saccharomyces cerevisiae , heterochromatin formation requires the Silent Information Regulator proteins, Sir2, Sir3 and Sir4 (refs 11 , 12 , 13 ). Assembly of Sir-dependent heterochromatin is believed to be a stepwise process in which silencing is initiated by binding of Sir4 to telomeres or the HM silent mating type loci via interactions with sequence-specific DNA-binding proteins, such as Rap1 (refs 11 , 14 ). Sir4 interacts directly with Sir2 (ref. 15 ), which is an NAD + -dependent histone deacetylase that targets lysine 16 of histone H4 (H4-K16) [16] . The Sir2-dependent deacetylation of H4-K16 promotes the subsequent nucleosome binding of the Sir3 protein [7] , [12] , [17] . Multiple cycles of histone deacetylation and Sir2, Sir3 and Sir4 binding are believed to control the spreading of the heterochromatic domain from the initial point of recruitment [10] , [11] , [13] , [15] . Both in vivo and in vitro studies indicate that Sir3 may be the primary structural component of yeast heterochromatin and that it can function, at least in part, independently of Sir2 and Sir4. For instance, overexpression of Sir3 can extend a domain of transcriptional silencing at telomeres in which Sir2 is largely absent and Sir4 is only detected at low levels [18] . Likewise, Sir3 overexpression allows formation of repressive heterochromatin at the HMR locus in a sir4-I1311N mutant that eliminates Sir4–Sir3 interactions [19] . In vitro , Sir3 binds to DNA and to nucleosomes, and the addition of Sir3 to recombinant nucleosomal arrays is sufficient to create a heterochromatin fibre that blocks early steps of homologous recombination in vitro [9] , [17] , [20] , [21] , [22] . Biochemical and genetic studies have led to the identification of a nucleosomal surface that plays a key role in Sir3 heterochromatin assembly. Notably, substitution of histone H4-K16 with a glutamine residue (H4-K16Q) eliminates the binding of Sir3 to heterochromatic loci in vivo , and mutations within Sir3 were identified as genetic suppressors of an H4-K16Q substitution allele [23] . Furthermore, the importance of H4-K16 for Sir3 nucleosomal recognition has been highlighted by several high-resolution structures of Sir3-nucleosome complexes [19] , [24] , [25] , [26] . These studies demonstrate that H4-K16 occupies a central cavity within the nucleosome-binding domain of Sir3, consistent with previous biochemical data showing that high affinity binding of Sir3 to histone peptides [27] and to mononucleosomes is disrupted by H4-K16 acetylation or glutamine substitution [9] , [28] . These results contrast with several in vitro studies indicating that Sir3 has a high nonspecific binding affinity for DNA [21] , [22] , and that the binding of Sir3 to 6-mer nucleosomal arrays is relatively insensitive to a H4-K16Q substitution [29] . Notably, these biochemical studies employed rather low-salt binding buffers that are likely to promote nonspecific DNA binding at the expense of specific nucleosomal interactions. Here, we describe ionic conditions that diminish the nonspecific DNA-binding activity of Sir3, resulting in binding to recombinant 12-mer nucleosomal arrays that is highly sensitive to the integrity of H4-K16. Using these conditions, we characterized the structure and subunit stoichiometry of Sir3 nucleosomal arrays by a combination of sedimentation velocity analytical ultracentrifguation (SV-AUC), atomic force microscopy (AFM) and a nucleosomal array capture assay. Notably, we have adapted a grid-based modelling method, called two-dimensional spectrum analysis (2DSA) [30] , coupled with a genetic algorithm (GA) and Monte Carlo (MC) analysis [31] , [32] , to fit sedimentation and diffusion parameters to the SV-AUC data. These modelling methods have allowed determination of both the native molecular weight and shape parameters of Sir3 nucleosomal arrays. Our results indicate that Sir3 binds to recombinant nucleosomal arrays at a stoichiometry of two Sir3 monomers per nucleosome, and that Sir3 binding leads to structures that are distinct from, and less compact than, canonical 30 nm fibres. Reconstitution of Sir3 nucleosomal arrays Our goal was to develop in vitro assay conditions in which Sir3 binding to nucleosomal arrays is highly sensitive to the substitution of histone H4-K16 with glutamine (H4-K16Q), a substitution that eliminates assembly of Sir heterochromatin in vivo [23] . To this end, nucleosomal arrays were reconstituted using recombinant wild-type (WT) or H4-K16Q histone octamers and DNA templates that contained 12 tandem copies of a nucleosome positioning sequence. Full-length Sir3 was purified from yeast and used in several binding assays. First, Sir3 binding was monitored by nucleosomal array capture ( Fig. 1a ). For this assay, a small concentration of octamers that contained a biotin group covalently attached to an engineered cysteine residue at the histone H2A C-terminus was added to chromatin, such that arrays contained approximately two biotinylated nucleosomes per 12-mer array. Sir3 was then bound to arrays in buffers containing increasing NaCl concentrations, arrays were captured on streptavidin magnetic beads and the amount of bound Sir3 was determined by western blot analysis. At low concentrations of NaCl (20 mM), Sir3 bound almost equivalently to the WT and H4-K16Q nucleosomal arrays, consistent with previous studies ( Fig. 1a ) [22] , [29] , [33] . In contrast, Sir3 bound almost exclusively to the WT arrays when the NaCl concentration was increased to 40–50 mM. Likewise, Sir3 strongly preferred the WT arrays when binding was performed in 20 mM sodium phosphate buffer (~40 mM Na + ; Supplementary Fig. 1 ). Furthermore, adding increasing amounts of Sir3 to WT and H4-K16Q arrays under these conditions showed saturation binding kinetics, with Sir3 binding to the WT arrays with an approximate maximum of two Sir3 monomers per nucleosome ( Fig. 1b ). In contrast, less than one monomer of Sir3 bound to each H4-K16Q nucleosome when assayed in 40 mM Na + buffer, even at high concentrations of Sir3 ( Fig. 1b ). 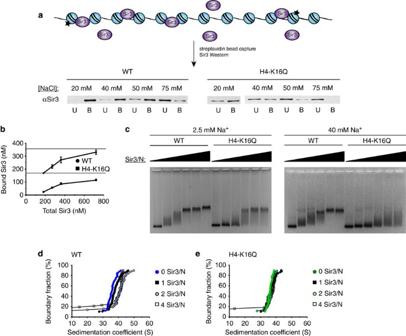Figure 1: Increased ionic strength buffer enhances the nucleosome-specific binding of Sir3. (a) Nucleosomal array capture and western blot analysis of Sir3 unbound (U) and bound (B) to WT and H4-K16Q arrays. (b) Quantification of bound versus unbound Sir3 to WT and H4-K16Q arrays of an experiment performed as inausing increasing Sir3 concentrations in 40 mM NaCl. (c) EMSA of Sir3 binding to WT and H4-K16Q 12-mer arrays in Tris containing 2.5 mM NaCl buffer (left) and phosphate buffer at ~40 mM Na+(right). Sir3/N is the number of Sir3 monomers per nucleosome positioning sequence, ranging from 0 to 8. (d,e) SV-AUC analyses. vHW plots of Sir3 binding to WT and H4-K16Q arrays, respectively. Sir3/N is the number of Sir3 monomers per nucleosome positioning sequence. Figure 1: Increased ionic strength buffer enhances the nucleosome-specific binding of Sir3. ( a ) Nucleosomal array capture and western blot analysis of Sir3 unbound (U) and bound (B) to WT and H4-K16Q arrays. ( b ) Quantification of bound versus unbound Sir3 to WT and H4-K16Q arrays of an experiment performed as in a using increasing Sir3 concentrations in 40 mM NaCl. ( c ) EMSA of Sir3 binding to WT and H4-K16Q 12-mer arrays in Tris containing 2.5 mM NaCl buffer (left) and phosphate buffer at ~40 mM Na + (right). Sir3/N is the number of Sir3 monomers per nucleosome positioning sequence, ranging from 0 to 8. ( d , e ) SV-AUC analyses. vHW plots of Sir3 binding to WT and H4-K16Q arrays, respectively. Sir3/N is the number of Sir3 monomers per nucleosome positioning sequence. Full size image Sir3 binding to 12-mer arrays was also monitored by an electrophoretic mobility shift assay (EMSA). As in the array capture assay in Fig. 1a , when assayed in low-salt Tris buffer (2.5 mM Na + ), Sir3 binding showed only a slight preference for WT versus H4-K16Q arrays ( Fig. 1c , left panel). Under these conditions, the addition of increasing quantities of Sir3 led to formation of heterogeneous, slow migrating complexes, as previously observed [22] , [29] , [33] . However, when binding reactions were performed in 20 mM sodium phosphate buffer (~40 mM Na + ), Sir3 demonstrated a strong preference for WT over H4-K16Q arrays ( Fig. 1c , right panel). Furthermore, under these conditions, increasing Sir3 concentrations led to the formation of a discrete complex of stable mobility. We next analysed Sir3 binding to arrays using SV-AUC. Phosphate buffer was used in these assays, as its Na + concentration (approximately 40 mM at pH 8.0) is within the ideal range of specific Sir3 binding (see Fig. 1a,c ), but unlike Tris buffer, phosphate does not absorb in the low ultraviolet range. In the absence of Sir3, both WT and H4-K16Q 12-mer nucleosomal arrays sedimented as fairly uniform species at ~34–36 S ( Fig. 1d,e ). Addition of Sir3 to the WT arrays shifted the distribution to larger S values, with maximal shifts at a ratio of two Sir3 monomers per nucleosome, leading to a structure that sedimented with a midpoint at ~42–45 S ( Fig. 1d ). A corresponding shift in S was not seen when Sir3 was added to H4-K16Q arrays ( Fig. 1e ), consistent with the binding specificity observed by both EMSA and array capture assays. In contrast to previous studies [22] , extensive aggregation or oligomerization was not observed when high concentrations of Sir3 were added to the arrays under these ionic conditions ( Fig. 1d ). Implementation of SV-AUC modelling The sedimentation behaviour of a macromolecule in an SV-AUC experiment is proportional to both its buoyant molecular weight and frictional properties governed by its overall shape. Consequently, the observed Sir3-induced changes in the S distribution of nucleosomal arrays in Fig. 1d could be due to an increased molecular weight, an altered conformation of the nucleosomal fibre, or a combination of both. To separate these two parameters, we applied a set of modelling methods implemented in UltraScan3 software, beginning with 2DSA, which uses a grid-based method to fit sedimentation and diffusion parameters to the SV-AUC data. The 2DSA analysis yields a set of solutes of specific sedimentation and diffusion properties that are likely to describe the experimental data set [30] . In order to distinguish between truly present solutes and false positives, a GA is used to refine the 2DSA solution [31] . GA is based on an evolutionary paradigm, using random cross-over, mutation and deletion events to alter the sedimentation and diffusion characteristics of the 2DSA solutes, and to eliminate false positive solutes by parsimonious regularization. The ultimate goal is to obtain a solution that satisfies Occam’s razor. According to Occam’s razor, from the many solutions possible for the lowest root-mean-square-deviation, the preferred solution is the one with the fewest solutes [34] . In such a solution, only solutes representing intrinsic sedimentation signal will remain. Finally, MC analysis of the GA solution is performed to further refine the fit and to obtain statistical descriptors of the final solutes [32] . This overall modelling process is termed 2DSA/GA-MC. When the partial specific volume is constant and known from other sources, the resulting solution gives fits for the sedimentation coefficient, partial concentration, molecular weight and frictional ratio ( f/f 0 ) of solutes present in the experimental sample. The f/f 0 value is the ratio of the frictional coefficient of an unknown molecule to the frictional coefficient of a perfect sphere of the same volume and density, and is thus a numerical descriptor of the particle’s anisotropy [35] . As the f/f 0 increases from 1.0, the molecule becomes more asymmetric, moving from spherical, to globular and then to rod-like, with most proteins falling between 1 and 4 (ref. 35 ). Although the 2DSA/GA-MC modelling approach has been successfully used to predict the molecular weight and shape of proteins and small nucleic acids, this method has not been previously applied to complex macromolecules, such as chromatin fibres. For an initial probe of this approach, 2DSA/GA-MC was employed to examine a DNA template containing 12 tandem copies of the 601 nucleosome positioning sequence separated by a 30-bp linker (601-177-12 DNA). van Holde Weischet (vHW) analysis of the SV-AUC data indicates that this ~2 kb DNA fragment sediments as a homogenous species of ~11 S ( Supplementary Fig. 2a ). In agreement with vHW analysis, 2DSA/GA-MC shows the presence of a single solute at 10.65 S ( Supplementary Fig. 2a,d ). The fit molecular weight of this solute also matched the predicted molecular weight (1.34 versus 1.31 MDa expected), and the f/f 0 ratio of 7.5 correctly indicated the presence of an extended rod ( Supplementary Fig. 2a,d ). As a further proof of principle, nucleosomal arrays were assembled with two concentrations of recombinant histone octamers to generate nucleosomal arrays that contained an average of ~6 or ~12 nucleosomes. Analysis of the SV-AUC data by either vHW analysis ( Supplementary Fig. 2b,c ) or 2DSA/GA-MC ( Supplementary Fig. 2b–d ) indicated the presence of relatively homogenous populations of solutes, and furthermore, the 2DSA/GA-MC modelling yielded reasonable fits for both the sedimentation coefficients ( S ) and the f/f 0 ratios. Likewise, the residuals for the 2DSA fits were largely random, indicating that this modelling method is appropriate for the analysis of chromatin fibres ( Supplementary Fig. 3a ). In contrast, the fit molecular weights, as determined by 2DSA/GA-MC, were much lower than the predicted molecular weights (1.17 versus 1.96 MDa and 2.3 versus 2.6 MDa). Likewise, 2DSA/GA-MC analysis of Sir3 nucleosomal arrays yielded molecular weights that were much smaller than expected (data not shown). Notably, an accurate determination of molecular weight by 2DSA/GA-MC analysis is dependent not only on the experimentally determined S and f/f 0 values, but also on the partial specific volume . is the solvated volume of a macromolecule, defined in millilitres per gram, and is essential for describing the hydrodynamic behaviour of molecules in solution [35] , [36] , [37] . The of proteins can be accurately predicted based on sequence and knowledge of the solvent components, however, there is no accurate method for predicting the of DNA or a complex of protein and DNA, which is also strongly dependent on the ionic strength of the solvent conditions [38] , [39] , [40] , [41] . UltraScan3 uses a weighted, average for protein–nucleic acid complexes, based on predicted stoichiometry ( is predicted to be 0.65 for 12-mer arrays). As SV-AUC experiments can only determine the buoyant molecular weight (MW), the value has a dominant role in absolute MW determination. Small changes in the parameter lead to considerable changes on the molecular weights determined by SV-AUC (ref. 38 ). These results indicate that analysis of chromatin fibres by 2DSA/GA-MC requires that the be experimentally determined. determination by density-contrast sedimentation We adapted a recently described method of experimentally measuring using SV-AUC that allows for the use of much less sample mass than traditional methods, such as measurement in a density balance [36] , [37] . In this method, samples are sedimented in three solvents containing either 0, 30 or 60% H 2 18 O. The resulting sedimentation coefficients are plotted as a function of solvent density, and the is calculated from the resulting plot (see Methods). We first applied this ‘density contrast’ method to a well-characterized protein, lysozyme, and to both a 177 bp DNA fragment and the 601-177-12 DNA template ( Supplementary Fig. 4 ). As expected, increasing concentrations of H 2 18 O led to a decrease in the sedimentation coefficients, and plotting the obtained S values against the solution density yielded experimental ’s that were remarkably similar to the predicted for both lysozyme and DNA. Indeed our experimental for lysozyme (0.726 ml g −1 ) is identical to the measured previously with a vibrating densitometer [42] . This density contrast method was then applied to nucleosomal arrays. First, a range of histone octamer concentrations were reconstituted on the 601-177-12 template to yield arrays with differing nucleosome density ( Fig. 2a ). Each sample was then subjected to density contrast sedimentation ( Supplementary Fig. 5 ), and the experimentally derived ’s are shown in Fig. 2 . Interestingly, as more nucleosomes were reconstituted onto the DNA, both the sedimentation coefficient and the increased in a linear relationship ( Fig. 2b,c ), indicative of both an increased molecular weight and an increased volume occupied by the chromatin fibre. Notably, the experimentally determined for the fully saturated, 35 S array (0.695 ml g −1 ) is consistent with the inverse of the previously determined buoyant density of chromatin fragments isolated from chicken cells (0.706 ml g −1 ) [43] . Importantly, the determinations were independent of the viscosity of the three separate solutions, and correcting the solutions for density led to vHW plots that overlayed closely, indicating that the sedimentation profiles of the samples in the three different buffers were highly reproducible ( Supplementary Fig. 6 ). 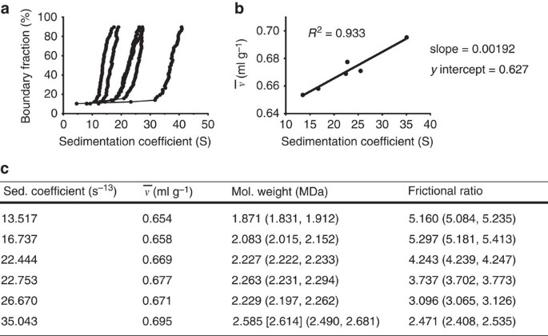Figure 2: The partial specific volume of variably saturated 601-177-12 nucleosomal arrays is directly proportional to the sedimentation coefficient. (a) vHW plots of 601-177-12 nucleosomal arrays at varying nucleosome saturation. (b) Theof the arrays in (a) plotted against their sedimentation coefficient.’s were determined inSupplementary Fig. 5. (c)Sandof arrays ina, and the molecular weight andf/f0ratio as determined by 2DSA/GA-MC, using experimentalnumbers determined inSupplementary Fig. 3. Numbers in parenthesis are 95% confidence intervals, and the number in brackets is the expected molecular weight for a 601-177-12 DNA template reconstituted with 12 histone octamers. Figure 2: The partial specific volume of variably saturated 601-177-12 nucleosomal arrays is directly proportional to the sedimentation coefficient. ( a ) vHW plots of 601-177-12 nucleosomal arrays at varying nucleosome saturation. ( b ) The of the arrays in ( a ) plotted against their sedimentation coefficient. ’s were determined in Supplementary Fig. 5 . ( c ) S and of arrays in a , and the molecular weight and f/f 0 ratio as determined by 2DSA/GA-MC, using experimental numbers determined in Supplementary Fig. 3 . Numbers in parenthesis are 95% confidence intervals, and the number in brackets is the expected molecular weight for a 601-177-12 DNA template reconstituted with 12 histone octamers. Full size image Experimentally determined ’s were used in 2DSA/GA-MC fits for each nucleosomal array sample ( Fig. 2c ). In striking contrast to our results with an estimated , the fit molecular weights increased in direct proportion with nucleosome saturation, from a molecular weight corresponding to a 12-mer template with approximately four nucleosomes (1.87 MDa), to one corresponding to a nearly saturated 12-mer array (2.59 MDa). In addition, as the DNA template wrapped around an increasing number of histone octamers, the f/f 0 ratio decreased, indicating the transition from an extended linear DNA molecule to a shorter, more globular chromatin fibre. This analysis was then applied to WT and H4-K16Q arrays assembled at a ratio of two Sir3 monomers per nucleosome ( Fig. 3 ). Density-contrast sedimentation was used to determine values from an average of three independent experiments (examples in Supplementary Fig. 7a,b ), and these values were used in 2DSA/GA-MC fitting of the SV-AUC data ( Fig. 3a,b ). 2DSA/GA-MC modelling indicated that WT and H4-K16Q nucleosomal arrays without Sir3 were similar in molecular weight, ~2.6 MDa, consistent with arrays containing ~12 nucleosomes on the 12mer template ( Fig. 3b ). Analysis of three independent WT and H4-K16Q arrays demonstrated remarkable reproducibility of the MW determinations (WT, 2.59±0.25 × 10 6 , H4-K16Q, 2.61±0.089 × 10 6 ). Likewise, these analyses yielded similar frictional coefficient ratios ( f/f 0 ), consistent with similar structures between WT and H4-K16Q arrays (WT, 2.16±0.19; H4-K16Q, 2.16±0.24). On addition of Sir3, the molecular weight of the WT fibre increased significantly, corresponding to the binding of ~24 monomers of Sir3 per nucleosomal array ( Fig. 3b ). Analysis of three independent Sir3 array reconstitutions support a stoichiometry of 21±4 molecules of Sir3 per nucleosome, consistent with an average ratio of ~2 monomers per nucleosome. In contrast, the addition of Sir3 to the H4-K16Q array did not lead to a significant shift in molecular weight ( Fig. 3b ). These data are fully consistent with Sir3-nucleosome stoichiometry measurements determined by the nucleosomal array capture assay ( Fig. 1b ), and they suggest that the 2DSA/GA-MC method can predict the molecular weight of complex protein–DNA complexes. 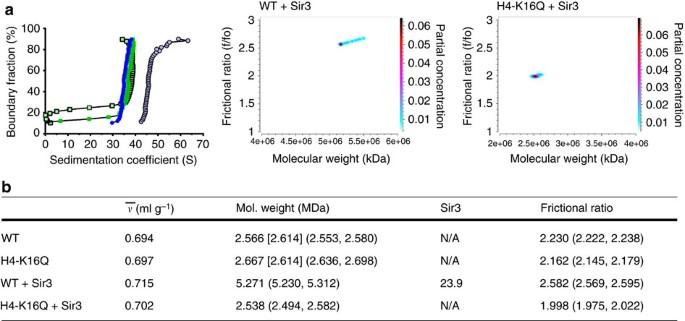Figure 3: Sir3 binds at two monomers per nucleosome and stabilizes the rod-like structure of chromatin. (a) Left panel, vHW of WT and H4-K16Q 12mer arrays ±2 Sir3 monomers per nucleosome. WT array is represented by dark blue closed circles, H4-K16Q by green closed squares, WT+Sir3 by light blue open circles and H4-K16Q+Sir3 by light green open squares. Middle and right panels, GA-MC plots showingf/f0versus molecular weight for WT and H4-K16Q with Sir3. (b) 2DSA/GA-MC data of samples inausing experimentally determinedvalues (seeSupplementary Fig. 7for examples). Numbers in brackets represent the expected molecular weight of a 601-177-12 array, and numbers in parentheses are 95% confidence intervals. Sir3 stoichiometry was calculated by subtracting the molecular weight of the array from the molecular weight of the array containing Sir3, divided by the molecular weight of 3xFLAG-tagged Sir3 (113 kDa). Figure 3: Sir3 binds at two monomers per nucleosome and stabilizes the rod-like structure of chromatin. ( a ) Left panel, vHW of WT and H4-K16Q 12mer arrays ±2 Sir3 monomers per nucleosome. WT array is represented by dark blue closed circles, H4-K16Q by green closed squares, WT+Sir3 by light blue open circles and H4-K16Q+Sir3 by light green open squares. Middle and right panels, GA-MC plots showing f/f 0 versus molecular weight for WT and H4-K16Q with Sir3. ( b ) 2DSA/GA-MC data of samples in a using experimentally determined values (see Supplementary Fig. 7 for examples). Numbers in brackets represent the expected molecular weight of a 601-177-12 array, and numbers in parentheses are 95% confidence intervals. Sir3 stoichiometry was calculated by subtracting the molecular weight of the array from the molecular weight of the array containing Sir3, divided by the molecular weight of 3xFLAG-tagged Sir3 (113 kDa). Full size image Sir3 binds to nucleosomal arrays as a monomer or dimer Several previous studies have shown that Sir3 forms oligomers in solution [27] , [33] , [44] , [45] , [46] . Sir3 contains a dimerization domain at its C-terminus [44] , [46] , and measurements of Sir3–Sir3 interactions indicates that Sir3 interacts with itself with low nanomolar affinity [27] , [44] . Our Sir3-nucleosome stoichiometry measurements are consistent with either the independent binding of two Sir3 monomers or the binding of a preformed Sir3 dimer. To evaluate the oligomeric state of Sir3 at the concentrations and buffer conditions employed here, SV-AUC analyses were performed. When analysed in phosphate buffer (~40 mM Na + ) at 171 nM protein (the same concentration used in Fig. 3 ), Sir3 was clearly heterogeneous, with at least two species apparent from the vHW distribution ( Supplementary Fig. 8a ). Analysis of the SV-AUC data by 2DSA/GA-MC modelling indicates that Sir3 is composed of a mixture of a monomer species that sediments at ~5 S and a population of dimers that sediment at ~8 S ( Supplementary Fig. 8a,b ). Furthermore, this distribution was not altered when Sir3 was analysed in phosphate buffer containing 150 mM Na + ( Supplementary Fig. 9a ). These data suggest that Sir3 may bind to each nucleosome within the array as either two monomers that subsequently dimerize or as a preformed dimer. Sir3 chromatin fibres are less condensed than 30 nm fibres The combination of density contrast sedimentation and 2DSA/GA-MC modelling yields two parameters, and f/f 0 ratio, that describe the shape of a macromolecule. In order to test whether these parameters can describe chromatin folding events, nucleosomal arrays were sedimented in the presence or absence of MgCl 2 , which promotes folding of an extended 12-mer array into structures resembling 30 nm chromatin fibres [47] , [48] . Samples were analysed in both low-salt (2.5 mM Na + ) Tris buffer and 20 mM phosphate (~40 mM Na + ) buffer conditions. Consistent with previous studies, addition of low concentrations of MgCl 2 to 12-mer arrays promoted formation of fibres that sediment at ~55 S ( Fig. 4a,b ). Density contrast sedimentation was used to determine values in all buffer conditions from three independent experiments (examples in Supplementary Fig. 7c,d ), and the SV-AUC data were analysed by 2DSA/GA-MC ( Fig. 4a–c ). Strikingly, Mg ++ -dependent folding was associated with an increased asymmetry of the fibres (that is, higher f/f 0 ratio) and a dramatic decrease in the solvated volume (that is, lower ; Fig. 4c ). These altered biophysical parameters are consistent with a Mg ++ - dependent transition from a flexible chromatin array to a more asymmetric, condensed chromatin fibre. Importantly, the fit molecular weights for the extended and folded samples were quite similar, demonstrating that 2DSA/GA-MC can distinguish contributions to S resulting from changes in shape versus changes in molecular weight. 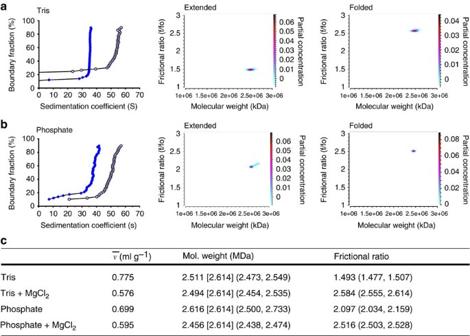Figure 4: 2DSA/GA-MC can distinguish between the shape and molecular weights of 10 nm and 30 nm fibres. (a) Left panel, vHW analysis of a saturated nucleosomal array in low-salt Tris buffer and in 1 mM MgCl2folding buffer. The extended sample is represented by closed blue circles, and the sample in folding buffer by open light blue circles. Middle and right panels, GA-MC plots off/f0versus molecular weight for extended and folded samples. (b) Same as ina, using samples prepared in phosphate buffer containing~40 mM Na+(extended), and in this buffer supplemented with 8 mM MgCl2(folded). (c) GA-MC data of samples inaandbusing experimentally determinedvalues (for examples, seeSupplementary Fig. 7). Number in brackets is the expected molecular weight of a 12mer array, and numbers in parentheses are 95% confidence intervals. Figure 4: 2DSA/GA-MC can distinguish between the shape and molecular weights of 10 nm and 30 nm fibres. ( a ) Left panel, vHW analysis of a saturated nucleosomal array in low-salt Tris buffer and in 1 mM MgCl 2 folding buffer. The extended sample is represented by closed blue circles, and the sample in folding buffer by open light blue circles. Middle and right panels, GA-MC plots of f/f 0 versus molecular weight for extended and folded samples. ( b ) Same as in a , using samples prepared in phosphate buffer containing~40 mM Na + (extended), and in this buffer supplemented with 8 mM MgCl 2 (folded). ( c ) GA-MC data of samples in a and b using experimentally determined values (for examples, see Supplementary Fig. 7 ). Number in brackets is the expected molecular weight of a 12mer array, and numbers in parentheses are 95% confidence intervals. Full size image Addition of Sir3 to 12-mer arrays (two monomers per nucleosome) led to small changes in both the parameter and the f/f 0 ratio ( Fig. 3b ). The asymmetry of the Sir3 chromatin fibres was quite similar to the Mg ++ -induced structures ( f/f 0 ratio of 2.54±0.19, n =4) and the values were larger than the WT arrays in the same phosphate buffer (2.16±0.19, n =6). Interestingly, the solvated volume ( ) did not decrease, as observed for Mg++-induced condensation, but rather it increased slightly (0.694–0.715 ml g −1 ). Notably, these changes in the or f/f 0 parameters were not observed when Sir3 was added to the H4-K16Q arrays ( Fig. 3b ). These data indicate that the binding of Sir3 to nucleosomal arrays leads to an asymmetric structure that is distinct from, and less condensed, than a Mg ++ -induced, 30 nm fibre. Visualization of Sir3 arrays by AFM To assess independently the structure of Sir3 chromatin fibres, samples were analysed by AFM ( Fig. 5 ). In low-salt Tris buffer (2.5 mM Na + ), WT arrays were highly extended, with an average height of 1.91 nm, consistent with a previous study indicating a height of ~2 nm for nucleosomes without linker histone [49] . The same arrays in 20 mM sodium phosphate buffer (~40 mM Na + ) were partially folded as expected in buffer with a moderate concentration of monovalent cation, with average heights of 1.60 and 1.84 nm for WT and H4-K16Q, respectively ( Fig. 5a,b ). In agreement with the SV-AUC data, the addition of Mg ++ led to formation of highly compact nucleosomal arrays with an average height of 5.62 nm ( Fig. 5a ). In contrast, addition of Sir3 to WT 12-mer arrays in phosphate buffer (~40 mM Na + ) led to formation of rod-like structures with an average height of 2.79 nm, whereas Sir3 addition to H4-K16Q arrays maintained a partially compacted structure with an average height of 1.72 nm ( Fig. 5c ). Similar results were obtained when Sir3 was incubated with arrays in phosphate buffer that contained 150 mM Na + ( Supplementary Fig. 9b,c ). Detailed images indicate that the Sir3 chromatin fibre is more compact than the array without Sir3, but these fibres have a more linear structure than the Mg ++ -compacted fibres (compare Fig. 5d,f ). 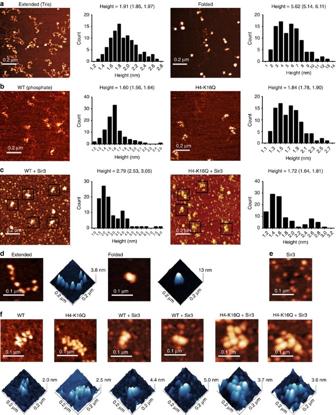Figure 5: Sir3 heterochromatin arrays are less compact than 30 nm fibres. (a) AFM images and height measurements of arrays in Tris (extended) and in Tris with 1 mM MgCl2(folded). The mean heights and 95% confidence intervals are shown above the height histograms. (b) Images and height histograms as inaof WT and H4-K16Q arrays in phosphate buffer. (c) Images and height histograms as inaof WT and H4-K16Q arrays in phosphate buffer with Sir3. Structures in black boxes are arrays bound or unbound by Sir3. (d) Representative, detailed 2D and 3D images of extended and folded arrays in low-salt Tris buffer. (e) Representative, detailed image of Sir3 protein alone. (f) Representative, detailed 2D and 3D images of WT and H4-K16Q arrays in phosphate±Sir3. Note that AFM heights are generally less than crystallographic values (but proportional to them) because of sample compression, adsorption of ions and small molecules on the substrate adjacent to the complexes being measured and chemical interactions between the probe and molecules. Figure 5: Sir3 heterochromatin arrays are less compact than 30 nm fibres. ( a ) AFM images and height measurements of arrays in Tris (extended) and in Tris with 1 mM MgCl 2 (folded). The mean heights and 95% confidence intervals are shown above the height histograms. ( b ) Images and height histograms as in a of WT and H4-K16Q arrays in phosphate buffer. ( c ) Images and height histograms as in a of WT and H4-K16Q arrays in phosphate buffer with Sir3. Structures in black boxes are arrays bound or unbound by Sir3. ( d ) Representative, detailed 2D and 3D images of extended and folded arrays in low-salt Tris buffer. ( e ) Representative, detailed image of Sir3 protein alone. ( f ) Representative, detailed 2D and 3D images of WT and H4-K16Q arrays in phosphate±Sir3. Note that AFM heights are generally less than crystallographic values (but proportional to them) because of sample compression, adsorption of ions and small molecules on the substrate adjacent to the complexes being measured and chemical interactions between the probe and molecules. Full size image Sir3 contains a BAH (Bromo-Associated Homology) domain within its N-terminus that binds to the nucleosomal surface that includes histone H4-K16 (refs 17 , 24 , 50 ). Several studies have demonstrated that Sir3 also contains a dimerization domain within its C-terminus, and that dimerization plays an essential role in assembly of heterochromatin [27] , [44] , [46] . Indeed, as expected, the isolated Sir3 BAH domain is entirely monomeric in phosphate buffer, sedimenting at 2.22 S ( Supplementary Fig. 10a,b ). To investigate whether Sir3 dimerization impacts the structure of Sir3 chromatin fibres, WT and H4-K16Q nucleosomal arrays were reconstituted with increasing amounts of the isolated Sir3 BAH domain ( Fig. 6 ) and array structure was analysed by AFM. As the Sir3 BAH domain was titrated to ten molecules per nucleosome (where optimal binding was seen), the arrays retained an extended conformation with linkers between each nucleosome still apparent. Interestingly, the average height of the WT arrays increased from 1.62 to 3.05 nm following Sir3-BAH binding ( Fig. 6a ). This value compares well to 2.79–3.29 nm for arrays containing full-length Sir3 ( Fig. 5c and Supplementary Fig. 9c ). These data suggest that the increase in nucleosomal height seen upon full-length Sir3 binding is primarily a result of the Sir3-BAH domain binding to the nucleosomal surface, whereas dimerization via the Sir3 C-terminal domain appears to promote nucleosome–nucleosome interactions that occlude linker DNA. 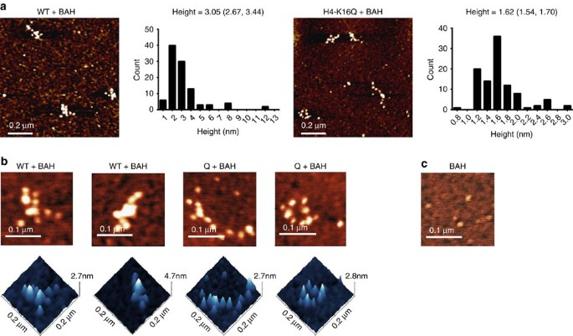Figure 6: The Sir3 BAH domain binds nucleosomes but does not coat or occlude linker DNA. (a) AFM images and height measurements of WT and H4-K16Q arrays bound by the Sir3 BAH domain. The mean heights and 95% confidence intervals are shown above the height histograms. (b) Representative, detailed 3D and 3D images of WT and H4-K16Q arrays in the presence of the Sir3 BAH domain in both 2D and 3D. Figure 6: The Sir3 BAH domain binds nucleosomes but does not coat or occlude linker DNA. ( a ) AFM images and height measurements of WT and H4-K16Q arrays bound by the Sir3 BAH domain. The mean heights and 95% confidence intervals are shown above the height histograms. ( b ) Representative, detailed 3D and 3D images of WT and H4-K16Q arrays in the presence of the Sir3 BAH domain in both 2D and 3D. Full size image In Saccharomyces cerevisiae , heterochromatin formation is mediated by the Sir proteins, which deacetylate nucleosomes at telomeres and silent mating type loci and assemble a chromatin fibre that results in the transcriptional and recombinational silencing of these regions [12] . Previous biochemical studies have disagreed both as to the nature of this repressive structure as well as to the stoichiometry of Sir proteins necessary for its formation [9] , [17] , [22] , [33] . Here, we have found that by transitioning to a buffer system with a moderate amount of monovalent cation, we are able to shield Sir3 from nonspecific interactions with DNA. Consequently, our assay conditions result in a heterochromatin fibre of discrete composition, which is highly sensitive to the integrity of H4-K16, a hallmark of yeast heterochromatin. By adapting the 2DSA/GA modelling algorithms, we have taken full advantage of analytical ultracentrifugation to describe both the native molecular weight and conformation of Sir3 chromatin fibres. Coupled with AFM and chromatin-binding analyses, our results indicate that Sir3 binds to model nucleosomal arrays with a stoichiometry of two monomers of Sir3 per nucleosome and that Sir3 creates a chromatin fibre that is distinct from and less compact than fibres condensed with divalent cations. SV-AUC experiments provide information about the conformational states of particles in solution, but can be difficult to interpret in situations where binding events may lead to conformational changes. By using 2DSA/GA-MC modelling to fit molecular weight and frictional properties to SV-AUC data, we were able to separate contributions to S derived from changes in size and changes in asymmetry. Although these modelling methods have been used successfully for analysing the sedimentation parameters of simple proteins and small nucleic acids, our study was the first to apply this approach to the analysis of chromatin fibres. During our initial studies, it was found that experimental determination of the parameter was essential for the 2DSA/GA-MC method to provide accurate determinations for the molecular weight of chromatin fibres. Using a density contrast approach, we found that the parameter, which is a measure of the solvated volume of a macromolecule, increased in direct proportion to the number of nucleosomes assembled on a template DNA. Furthermore, the provided a measurement of the shape of a chromatin fibre, as it decreased dramatically as an extended nucleosomal array folded into a 30-nm fibre (that is, due to Mg ++ ). Surprisingly, the of a nucleosomal array that was bound by 24 molecules of Sir3 did not change dramatically, which, in combination with AFM imaging, provided further evidence that Sir3 does not induce extensive nucleosomal array condensation but rather may ‘coat’ the chromatin fibre while occluding linker DNA. In WT yeast, the Sir2, Sir3 and Sir4 proteins co-localize at heterochromatin domains, and biochemical studies have demonstrated high affinity interactions between each of the Sir proteins [27] . In yeast whole-cell extracts, however, the majority of Sir3 is not associated with either Sir2 or Sir4, whereas Sir2 and Sir4 form a stable complex [15] . Notably, a Sir2/Sir3/Sir4 complex can be assembled with recombinant proteins, either by combining the purified Sir2/Sir4 complex and Sir3, or by co-overexpression in baculovirus-infected cells [15] , [29] , [51] . Surprisingly, however, the Sir2/Sir3/Sir4 complex formed in solution binds with nearly equal affinity to acetylated nucleosomes or nucleosomes harbouring H4-K16Q [29] . Thus, it is unclear whether this complex interacts with chromatin in a physiologically relevant manner. Recently, it was suggested that a preassembled Sir2/Sir3/Sir4 complex might play a role in the initial establishment stage of heterochromatin formation, and that the subsequent assembly and spreading of Sir proteins may require an ordered, stepwise assembly pathway [52] . In this model, the initial binding of an intact Sir2/Sir3/Sir4 complex to silencing regions via interactions with sequence-specific DNA-binding factors would promote deacetylation of H4-K16 on an adjacent nucleosome. This would lead to binding of Sir3 to the nucleosome, which would then facilitate binding of a Sir2–Sir4 complex that would deacetylate an adjacent nucleosome and repeat the cycle. Interestingly, both Sir3 and Sir4 bind to DNA, and each also binds to similar or overlapping histone surfaces with high affinity [27] , [28] , including the histone residues flanking H4-K16. Likewise, Sir2 must also interact with this region of the H4 N-terminus during histone deacetylation, and must then dissociate before Sir3 binding. These complex binding interactions support the view that a stepwise assembly mechanism may be required to ensure assembly of a bona fide heterochromatin fibre. Several studies have demonstrated that Sir3 contains a dimerization domain within its C-terminus, and that dimerization plays an essential role in the assembly of heterochromatin [27] , [44] , [45] , [46] . Although, Sir3 forms dimers and higher oligomers at high protein concentrations [45] , we found that Sir3 is present primarily as a mixture of monomers and dimers at concentrations used for heterochromatin assembly in vitro (<200 nM) and in buffers containing 40–150 mM Na + . Together with our stoichiometry measurements, these data suggest a model in which two monomers of Sir3 bind to a single nucleosome, with each BAH domain of Sir3 occupying the nucleosomal surface exemplified by H4-K16. In this model, the antiparallel nature of the Sir3 dimerization domain could then facilitate interactions between neighbouring nucleosomes ( Fig. 7 ). This model is consistent with our AFM imaging of nucleosomal arrays bound by the isolated BAH domain that shows a ‘balls-on-a-string’ structure rather than the more homogenous, elongated fibre observed for WT Sir3. The known interaction of Sir4 with the Sir3 C-terminal domain might also direct a Sir2–Sir4 complex to bridge adjacent nucleosomes. Interestingly, the binding of Sir2/Sir4 to the linker region is consistent with a previous prediction of the stoichiometry of a Sir2/Sir3/Sir4 complex bound to a 6-mer array [33] . 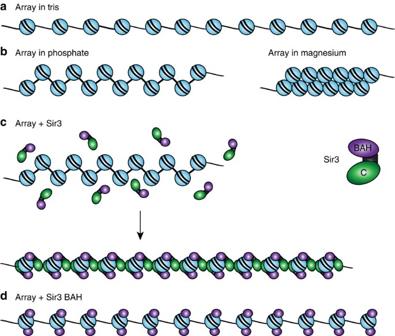Figure 7: Model for a Sir3 chromatin fibre. (a) Diagram of a 12-mer array in low-salt Tris buffer. (b) Arrays in 20 mM phosphate buffer pH 8.0 (containing ~40 mM Na+) are partially folded. Arrays in 1 mM MgCl2buffer fold into 30 nm fibres. (c) Sir3 binds to arrays as a monomer, then subsequent dimerization via the Sir3 c-terminus bridges neighbouring nucleosomes. Sir3 dimerization leads to array compaction distinct from 30 nm folding. (d) The Sir3 BAH domain binds to nucleosomes but cannot occlude linker DNA because of the absence of the C-terminal dimerization domain. Figure 7: Model for a Sir3 chromatin fibre. ( a ) Diagram of a 12-mer array in low-salt Tris buffer. ( b ) Arrays in 20 mM phosphate buffer pH 8.0 (containing ~40 mM Na + ) are partially folded. Arrays in 1 mM MgCl 2 buffer fold into 30 nm fibres. ( c ) Sir3 binds to arrays as a monomer, then subsequent dimerization via the Sir3 c-terminus bridges neighbouring nucleosomes. Sir3 dimerization leads to array compaction distinct from 30 nm folding. ( d ) The Sir3 BAH domain binds to nucleosomes but cannot occlude linker DNA because of the absence of the C-terminal dimerization domain. Full size image The Mg ++ -dependent folding of model 12-mer nucleosomal arrays creates a two-start helical fibre with a diameter of ~30 nm (ref. 53 ). We find that this condensation reaction is accompanied by a large decrease in the solvated volume of the fibre as well as an increase in asymmetry of the array. Furthermore, AFM analysis confirms the formation of a fibre with a greatly increased height compared with an unfolded array. In contrast, addition of Sir3 to a nucleosomal array leads to little change in the solvated volume, although the Sir3 chromatin fibre is more asymmetric than arrays that lack Sir3. AFM analyses also indicate that Sir3 creates a linear structure that is less extended than the unbound nucleosomal array, but also more rod-like and rigid. Interestingly, a model in which Sir3 monomers bridge adjacent nucleosomes closely resembles the crystal packing interactions observed for a Sir3-nucleosome X-ray structure [24] , and it is consistent with EM images demonstrating long linear filaments of Sir proteins bound to yeast chromatin [17] . This linear model of heterochromatin structure is in stark contrast to the existing dogma that heterochromatin is composed of tightly compacted chromatin fibres [2] . Instead, it suggests that heterochromatin proteins function by stabilizing interactions between underlying nucleosomes and DNA, and by serving as a physical barrier to the actions of chromatin remodelling enzymes. Proteins Lysozyme from chicken egg white was obtained from Sigma-Aldrich as a 10 mg ml −1 solution, and dialysed into 20 mM sodium phosphate buffer pH 8.0. Final concentration was determined via spectroscopy. FLAG-tagged Sir3 protein was overexpressed and affinity purified from yeast [9] , [10] . Briefly, yeast cultures transformed with a plasmid containing 3xFLAG-tagged Sir3 under a galactose-inducible promoter were grown to optical density (OD) 0.6 and induced with 2% galactose for 8 h. Cultures were pelleted, resuspended in E Buffer (20 mM HEPES pH 7.4, 350 mM NaCl, 10% glycerol, 0.1% Tween-20 and protease inhibitors) and frozen in liquid nitrogen. Pellets were ground using a cold mortar and pestle with frequent additions of liquid nitrogen until approximately 50% of cells appeared lysed under a microscope. Cells were incubated on ice in E buffer for 30 min, then spun at 3,000 r.p.m. for 15 min to remove debris. Supernatant was clarified at 40,000 r.p.m. for 1 h, then the aqueous layer was removed from the lipid layer using a syringe. Lysate was incubated with anti-Flag resin (Sigma-Aldrich) for 3 h at 4 °C. Resin was washed in E buffer, then Sir3 was eluted in batch via four 30 min incubations of resin with E Buffer containing 100 μg ml −1 3xFLAG peptide (Sigma-Aldrich). Concentration was determined by comparison to known concentrations of BSA electrophoreses on the same Coomassie-stained SDS–polyacrylamide gel electrophoresis (PAGE) gel. 6xHis-tagged Sir3 D205N BAH was expressed in Rosetta cells and purified using Qiagen Ni-NTA resin (Qiagen) according to the manufacturer’s protocol. It was quantified spectroscopically using an extinction coefficient predicted by UltraScan3 software (40,090 OD/mol*cm). Recombinant Xenopus laevis histones were expressed in BL21 cells, purified and assembled into histone octamers according to the standard protocols [54] . Biotinylated octamers contained a H2A derivative where serine 113 was changed to a cysteine. H2A-S113C-containing octamers were dialysed into biotinylation buffer (35 mM Tris pH=7.4, 1 mM EDTA, 2 M NaCl) and reacted at 20 μM octamer with 800 μM Maleimide-PEG2-Biotin (Thermo Fisher Scientific Inc., Cat# 21902; dry powder reconstituted immediately before use into biotinylation buffer). Reaction proceeded on ice for 48 h. DNA The 601-177-12 nucleosomal array template containing 12 copies of the Widom 601 nucleosome positioning sequence was digested from its plasmid backbone using EcoRV and purified by size-exclusion chromatography. 601-177-1 DNA was generated by digestion of the 601-177-12 template with Sca I. DNA fragments were dialysed into 20 mM sodium phosphate pH 8.0 before SV-AUC. Nucleosomal array assembly Nucleosomal arrays were assembled by combining recombinant histone octamers and 601-177-12 DNA template at varying molar ratios of octamer to nucleosome positioning sequence in 2 M NaCl, and stepwise salt dialysis was performed until completion into either 2.5 mM NaCl and TE, or 20 mM sodium phosphate pH 8.0 with 0.1 mM EDTA. Arrays are in phosphate buffer unless otherwise indicated. Array saturation was determined by Sca I digestion followed by analysis via native PAGE and by SV-AUC. To construct partially biotinylated nucleosomal arrays, WT and biotinylated octamers were mixed at an 85:15 molar ratio and reconstituted as above, using the 208-12 DNA template. Nucleosomal array capture Biotinylated nucleosomal array of 16 nM concentration (192 nM nucleosomes) was bound to 384 nM Sir3p (unless experimentally varied) in pulldown buffer (35 mM Tris pH 7.4, 50 mM NaCl unless experimentally varied, 1.75 mM MgCl2, 0.05% Tween-20, 1 mM DTT) for 25 min at 22 °C. For Supplementary Fig. 1 , 20 mM sodium phosphate buffer pH 8.0 was used in place of pulldown buffer. This reaction was then bound to 10 μg μl −1 Streptavidin-coated magnetic beads (Invitrogen, Cat# 11205D) for 5 min at 22 °C. The magnetic beads had been washed twice in pulldown buffer and blocked for 15 min at 22 °C in pulldown buffer supplemented with 100 μg ml −1 BSA. During blocking and array binding, beads were kept continually suspended by gentle rotation. After binding, the beads were magnetically captured and the supernatant ‘unbound’ fraction was removed. The beads were resuspended in 1 × SDS–PAGE sample buffer, heated for 5 min at 95 °C, and care was taken to magnetically extract the stripped beads from the supernatant ‘bound’ fraction. These fractions were subjected to SDS–PAGE, electroblotted onto nitrocellulose and detected by HRP-FLAG (1:5,000, Sigma-Aldrich, Cat# A8592) immunoblotting. EMSA 300 ng WT or H4-K16Q nucleosomal array in Tris buffer containing 2.5 mM NaCl or phosphate buffer containing approximately 40 mM Na + was combined with Sir3 at a range of 0–8 monomers per nucleosome to a final concentration of 10 ng μl −1 array and 5% glycerol. Binding reactions were incubated at room temperature for 30 min, run on 1% TBE agarose gels and stained with ethidium bromide. SV-AUC SV-AUC was carried out using 400 μl sample loaded into two-sector Epon centerpieces in an An60 Ti rotor in a Beckman Optima XL-I analytical ultracentrifuge, and run at 20 °C. Measurement was completed in intensity mode. Nucleosomal arrays were run at 10 ng μl −1 concentrations with the indicated amount of Sir3 or MgCl 2 at 20,000 r.p.m., and were measured at 215 nm (for arrays in phosphate buffer) or 260 nm (for samples containing Tris or Sir3). Lysozyme was loaded to an OD of 0.4, and run at 41,000 r.p.m. and measured at 280 nm. DNA fragments were run at 10 ng μl −1 in phosphate buffer with 300 mM NaCl added to reduce concentration-dependent nonideality, and measured at 260 nm. The 601-177-12 fragment was run at 30,000 r.p.m. and the 601-177-1 fragment at 48,000 r.p.m. Sir3 alone was run in the indicated solution at 171 nM and 40,000 r.p.m. and measured at 215 nm, and Sir3 BAH alone was run at 1.71 μM and 48,000 r.p.m. For determination, three preparations of sample were run as above, with 0, 30 or 60% H 2 18 O (obtained from Cambridge Istotope Laboratories) added in place of H 2 16 O. The obtained S values were then plotted as a function of solvent densities, linear regression was performed and the was calculated by dividing the slope of the resulting line by the y -intercept. Solvent densities and viscosities were obtained from the literature [36] . Linear regression was performed using GraphPad Prism software. 2DSA/GA-MC All SV-AUC data were analysed using UltraScan3 software, version 2.1 and release 1706 (ref. 55 ) and fitting procedures were completed on XSEDE clusters at the Texas Advanced Computing Center (Lonestar, Stampede) and at the San Diego Supercomputing Center (Trestles) through the UltraScan Science Gateway ( https://www.xsede.org/web/guest/gateways-listing ). Raw intensity data were converted to pseudo-absorbance by using the intensity of the air above the meniscus as a reference and edited. Next, 2DSA was performed to subtract time-invariant noise and the meniscus was fit using ten points in a 0.05-cm range. Arrays were fit using an S range of 5–60 S , an f/f 0 range of 1–10 with 64 or 100 grid points for each, 10 uniform grid repetitions and 400 simulation points. 2DSA was then repeated at the determined meniscus to fit radially invariant and time-invariant noise together using five iterations. vHW analysis was completed using these noise subtraction profiles to determine S . Where indicated, GA was initialized by binning major solutes in the 2DSA data set, and run via LIMS. Major solutes from GA analysis were then binned and run again using GA with 50 MC iterations. AFM For AFM experiments, an Agilent AFM 5500 instrument (Agilent) and silicon nitride cantilevers were used (force constant=25–75 N m −1 , resonant frequency=332 kHz). Imaging was done in air using the acoustic AC mode with an amplitude of ~10 nm and a set-point reduction of about 10%, scanning at one line per second. Immobilization of chromatin arrays on mica surface was done as follows. First, 1 μl of Sir3 protein solution (39 ng μl −1 ) was added to the phosphate or Tris buffer (7 μl) followed by addition of 1 μl of chromatin array (10 ng μl −1 ) and mixed gently, maintaining a ratio of four Sir3 molecules/nucleosome. For Sir3 BAH D205N experiments, BAH was added at four (data not shown) and ten monomers per nucleosome as above. After 30 min, 0.5% glutaraldehyde solution (1 μl) was added to this mixture for crosslinking and incubated for 10 min. (3-Aminopropyl)triethoxysilane was deposited on freshly cleaved mica substrate using vapour deposition. The crosslinked chromatin solution was diluted to 1 ng μl −1 and 3 μl was added to this APTES-modified mica surface, and after 5 min, the surface was cleaned three times using 400 μl of buffer solution, dried carefully using argon gas and immediately used for imaging. To image only chromatin arrays, the first mixing step with Sir3 was omitted. How to cite this article: Swygert, S. G. et al. Solution-state conformation and stoichiometry of yeast Sir3 heterochromatin fibres. Nat. Commun. 5:4751 doi: 10.1038/ncomms5751 (2014).